Separation of a functional deubiquitylating module from the SAGA complex by the proteasome regulatory particle Gene expression is an intricate process tightly linked from gene activation to the nuclear export of mRNA. Recent studies have indicated that the proteasome is essential for gene expression regulation. The proteasome regulatory particle binds to the SAGA complex and affects transcription in an ATP-dependent manner. Here we report that a specific interaction between the proteasomal ATPase, Rpt2p and Sgf73p of the SAGA complex leads to the dissociation of the H2Bub1-deubiquitylating module (herein designated the Sgf73-DUBm) from SAGA both in vitro and in vivo . We show that the localization of the Sgf73-DUBm on chromatin is perturbed in rpt2-1 , a strain of Saccharomyces cerevisiae that is specifically defective in the Rpt2p-Sgf73p interaction. The rpt2-1 mutant also exhibits impaired localization of the TREX-2 and MEX67-MTR2 complexes and is defective in mRNA export. Our findings collectively demonstrate that the proteasome-mediated remodelling of the SAGA complex is a prerequisite for proper mRNA export. The 26S proteasome is a highly conserved protein-degrading machine composed of a barrel-shaped 20S core particle (CP) that is capped at each end with a 19S regulatory particle (RP) [1] . Whereas the 20S CP has protease activity, the base complex of the 19S RP exhibits chaperone-like activity in addition to proteolytic functions [2] , [3] . It has been reported that PA700, the mammalian homologue of the 19S RP, binds to misfolded protein substrates, represses their aggregation and remodels their conformation prior to proteolysis [4] , [5] , [6] . At the end of the M phase, the cyclin B and cdc2 subunits of cyclin B-Cdc2 kinase are separated by the 26S proteasome via a mechanism that does not require proteolysis of the cyclin B substate [7] . In addition, the base complex (that is, the hexameric ATPase component) of the 19S RP has been shown to be involved in gene expression irrespective of its proteolytic activity [8] , [9] . The non-proteolytic functions of the proteasome include its abilities to modulate ubiquitin-dependent covalent histone modifications [10] and remodel/stabilize the stalled polymerase complex to support efficient transcriptional elongation [11] . The functions of the 19S RP in transcriptional elongation are supported by the observed elongation defects in the yeast 19S RP ATPase mutant strains, SUG1 and SUG2 (refs 10 , 12 ). Recently, the 19S RP was suggested to regulate the assembly of the active transcription complex at the promoter [13] by facilitating the interactions between the Spt-Ada-Gcn5-acetyltransferase (SAGA, a yeast transcriptional coactivator) complex and promoter-bound transcription activators [14] . The same study demonstrated a physical interaction between the 19S RP and the SAGA complex and suggested that the 19S RP may change the biochemical properties of the SAGA complex. SAGA is a multisubunit complex of 1.8 MDa that coordinates multiple post-translational modifications of histones [15] to regulate diverse cellular functions, including the acetylation of histone H3 (ref. 16 ), the recruitment of the RNA polymerase II (RNA PolII) pre-initiation-complex and the deubiquitylation of histone H2B mono-ubiquitylation at lysine 123 (H2Bub1) [17] , [18] , [19] . Among the submodules of the SAGA complex, the deubiquitylating module (DUBm), which consists of the Sgf73, Ubp8, Sus1 and Sgf11 subunits [20] , [21] , is responsible for the deubiquitylation of H2Bub1 (refs 17 , 18 , 19 ). The DUBm facilitates elongation via the deubiquitylation of H2Bub1 (ref. 22 ) and contributes to other aspects of gene expression, such as gene gating and mRNA export [23] . Interestingly, previous studies have suggested that the proteasome may be involved in mRNA export [6] , [24] , [25] . For example, Sem1, a component of the 19S RP lid subcomplex, was identified as a functional subunit of the TREX-2 complex [26] , [27] . The physical interaction between the proteasome and the SAGA complex suggests that the proteasome may induce a conformational change in the SAGA complex through its ATP-dependent chaperone-like activity. Here we report a novel non-proteolytic function of the 19S RP: it specifically interacts with the SAGA complex to induce the dissociation of an Sgf73p-Ubp8-containing complex that displays deubiquitylation activity. Remodelling of the SAGA complex by the proteasome affects the association of the TREX-2 complex with the nuclear pore complex (NPC), which is essential for mRNA export. Our data further suggest that this proteasome-mediated alteration of the SAGA complex is involved in transcription-coupled mRNA export. The proteasomal ATPase Rpt2p specifically binds to Sgf73p Previous studies have demonstrated that there is a physical interaction between the 19S RP and the SAGA complex [28] . To investigate the nature of the interactions between the 19S RP and the SAGA complex subunits, we performed in vitro GST pull-down assays with purified SAGA and GST-fused components of the 19S RP. The SAGA complex bound specifically to Rpt2p ( Supplementary Fig. S1a , lane 2 versus lanes 1 and 3–6) but not Pre4p (a subunit of the 20S CP) or Rpn1-12p (non-ATPase 19S RP subunits) ( Supplementary Fig. S1a , lanes 7 and 8–18). A previous study on the interaction between the human Rpt2p homologue, S4, and the human Sgf73p homologue, Sca7 (ref. 29 ), suggested that Sgf73p may be a binding partner of Rpt2p. To test the potential binding relationship between Rpt2p and Sgf73p, we used GST pull-down assays with SAGA complexes from the wild-type ( wt ) and sgf73Δ strains. Our results indicated that Rpt2p specifically interacted with the wt SAGA complex in vitro ( Supplementary Fig. S1b , lane 3) but not with the SAGA complex lacking Sgf73p ( Supplementary Fig. S1b , lane 6 versus lane 9). As Sgf73p is a subunit of the DUBm, we tested whether other subunits of the DUBm could alter the interaction between Sgf73p and Rpt2p. GST pull-down assays showed that the Sgf73p-Rpt2p interaction patterns of ubp8Δ and sgf11Δ were similar to those observed in wt ( Supplementary Fig. S1b , lanes 9 and 12). Thus, the interaction between the 26S proteasome and the SAGA complex appears to occur specifically through Sgf73p and Rpt2p. We next sought to identify the Rpt2p-binding domain for the SAGA complex by performing GST pull-down assays with a series of truncated versions of Rpt2p. Our results revealed that the N-terminal domain, specifically the basic patch of Rpt2p (RKKRK), was responsible for binding the SAGA complex ( Supplementary Fig. S1c , lane 9). Based on this finding, we used a trans-replacement method to engineer an Rpt2p mutant lacking the RKKRK patch (designated rpt2-1 ). Collectively, these data show that the proteasomal ATPase, Rpt2p, specifically binds to Sgf73p of the SAGA complex. The 19S RP dissociates an Sgf73p-Ubp8p-containing complex Having shown that the interaction between the 19S RP and the SAGA complex is specific, we next investigated the possible effects of this interaction. We hypothesized that the 19S RP alters the conformation of the SAGA complex via the proteasome’s innate ATP-dependent chaperone-like activity [3] . To assess this, we combined purified Spt7-TAP-tagged SAGA complexes from rpt2-1 with proteasomes (26S or 19S) in the presence or absence of ATP. The SAGA complexes were then immobilized in calmodulin resin, and the bound and supernatant fractions were separated. Western blotting was performed with antibodies against CBP (Spt7p), FLAG (Sgf73p), MYC (Ubp8p) and HA (Gcn5p) ( Fig. 1 ). Sgf73p and Ubp8p were detected in the supernatant in the presence of ATP ( Figs. 1a, b , lane 4), whereas neither Gcn5p nor Spt7p was detected in the supernatant, regardless of the presence of ATP ( Fig. 1a,b , lanes 4 and 5). These data indicate that an Sgf73p-Ubp8p-containing complex is separated from the SAGA complex by the 19S RP in an ATP-dependent manner. Interestingly, both Sgf73p and Ubp8p are subunits of the DUBm. 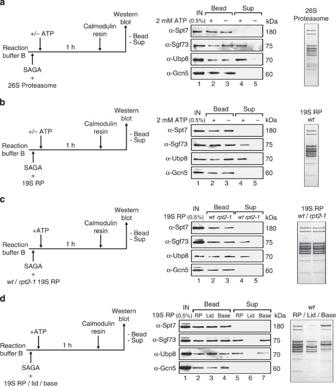Figure 1: The 19S RP separates a Sgf73p-Ubp8p-containing complex from the SAGA complex in an ATP-dependent manner. (a,b) Schematic diagram ofin vitroexperiments (left panel). Spt7-TAP-tagged SAGA complexes purified fromrpt2-1were combined with the 26S proteasome (a) and the 19S RP (b) purified fromwtin the presence or absence of 2 mM ATP. After reaction with calmodulin resin, the bound proteins and supernatants were eluted in SDS–PAGE sample buffer and analysed by western blotting with antibodies against CBP (Spt7p), FLAG (Sgf73p), MYC (Ubp8p) and HA (Gcn5p). (c,d) Schematic diagram ofin vitroexperiments (left panel). Experiments were performed as in (a), except that the Spt7-TAP-tagged SAGA complexes fromrpt2-1were combined with the 19S RP purified fromwtandrpt2-1(c) and the 19S RP, lid complex or the base complex fromwt(d). The bound proteins and supernatants were analysed using western blotting with antibodies against CBP (Spt7p), FLAG (Sgf73p), MYC (Ubp8p) and HA (Gcn5p). The purified 26S proteasome, 19S RP, lid complex and the base complex were visualized using Coomassie blue staining (right panel). Figure 1: The 19S RP separates a Sgf73p-Ubp8p-containing complex from the SAGA complex in an ATP-dependent manner. ( a , b ) Schematic diagram of in vitro experiments (left panel). Spt7-TAP-tagged SAGA complexes purified from rpt2-1 were combined with the 26S proteasome ( a ) and the 19S RP ( b ) purified from wt in the presence or absence of 2 mM ATP. After reaction with calmodulin resin, the bound proteins and supernatants were eluted in SDS–PAGE sample buffer and analysed by western blotting with antibodies against CBP (Spt7p), FLAG (Sgf73p), MYC (Ubp8p) and HA (Gcn5p). ( c , d ) Schematic diagram of in vitro experiments (left panel). Experiments were performed as in ( a ), except that the Spt7-TAP-tagged SAGA complexes from rpt2-1 were combined with the 19S RP purified from wt and rpt2-1 ( c ) and the 19S RP, lid complex or the base complex from wt ( d ). The bound proteins and supernatants were analysed using western blotting with antibodies against CBP (Spt7p), FLAG (Sgf73p), MYC (Ubp8p) and HA (Gcn5p). The purified 26S proteasome, 19S RP, lid complex and the base complex were visualized using Coomassie blue staining (right panel). Full size image Identical in vitro experiments using the 19S RP from rpt2-1 ( Fig. 1c ) showed that Sgf73p and Ubp8p were not detected in the supernatant ( Fig. 1c , lane 5). Thus, the protein–protein interaction between Sgf73p and Rpt2p appears to be important for the separation of the Sgf73p-Ubp8p-containing complex from the SAGA complex ( Fig. 1c , compare lanes 4 and 5). Whereas the barrel-shaped 20S CP consists of four stacked rings [30] , the 19S RP can be divided into two subcomplexes [31] : the base and the lid [32] . The base complex contains four non-ATPase subunits (Rpn1, −2, −10 and −13) and six AAA-type ATPases (Rpt1-6) that exhibit chaperone-like activity [3] . To identify the subcomplex(es) of the 19S RP that is/are responsible for the separation of the Sgf73p-Ubp8p-containing complex from the SAGA complex, we conducted in vitro experiments with the whole 19S RP, the lid and the base ( Fig. 1 , right panel). Our results revealed that the base complex alone, but not the lid complex alone, was sufficient to separate the Sgf73p-Ubp8p-containing complex from the SAGA complex ( Fig. 1d , lane 7). These data indicate that the 19S RP dissociates the Sgf73p-Ubp8p-containing complex from the SAGA complex in an ATP-dependent manner through a specific interaction with SAGA. The proteasome separates a functional Sgf73-DUBm from SAGA We speculated that the separation of the Sgf73p-Ubp8p-containing complex via a specific interaction of the proteasome with SAGA could affect the relative abundance of the Sgf73-DUBm in the SAGA complexes differently in wt versus rpt2-1 cells. First, we checked the integrity of the SAGA complexes in the wt and rpt2-1 strains, using silver staining of Spt7-TAP-tagged SAGA complexes purified from wt and rpt2-1 ( Fig. 2a ). Our results indicated that the SAGA complex is intact in rpt2-1 . 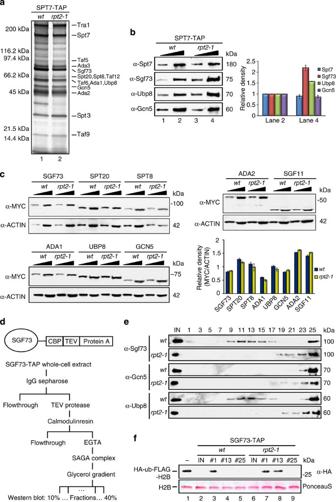Figure 2: The Sgf73p-DUBm separated from the SAGA complex has functional H2Bub1 deubiquitylation activityin vivo. (a) Spt7-TAP-tagged SAGA complexes fromwtandrpt2-1were purified using the TAP purification method67and visualized using silver staining. Protein molecular weight standards are indicated. (b) Twofold serially diluted samples of Spt7-TAP-tagged SAGA complexes purified fromwtandrpt2-1were analysed using western blotting with antibodies against CBP (Spt7p), FLAG (Sgf73p), MYC (Ubp8p) and HA (Gcn5p). The blots shown are representative of three independent experiments. Western blot signals were quantified using the Image J software (NIH), and standard deviations are shown by error bars. (c) MYC-taggedwtandrpt2-1cells were grown in YPD at 30 °C, and total cell extracts were analysed using SDS–PAGE and western blotting using a monoclonal anti-MYC antibody and an anti-ACTIN antibody (control). The quantified results and standard deviations are graphed in the right panel. Western blot signals were quantified using the Image J software (NIH), and standard deviations from four independent experiments are shown by error bars. (d) Schematic diagram ofin vitroexperiments. (e) Sgf73-TAP-tagged SAGA complexes purified fromwtandrpt2-1were fractionated by 10–40% glycerol gradient centrifugation, and the fractions were analysed using western blotting with antibodies against CBP (Sgf73p), MYC (Ubp8p) and HA (Gcn5p). IN, input. (f)In vitrodeubiquitylation assays of three glycerol gradient fractions (fractions 1, 13 and 25) were conducted using HA-ub-FLAG-H2B as the substrate. Western blotting was performed with an antibody against HA. Mock-treated H2Bub1 substrate was used as the input. Figure 2: The Sgf73p-DUBm separated from the SAGA complex has functional H2Bub1 deubiquitylation activity in vivo . ( a ) Spt7-TAP-tagged SAGA complexes from wt and rpt2-1 were purified using the TAP purification method [67] and visualized using silver staining. Protein molecular weight standards are indicated. ( b ) Twofold serially diluted samples of Spt7-TAP-tagged SAGA complexes purified from wt and rpt2-1 were analysed using western blotting with antibodies against CBP (Spt7p), FLAG (Sgf73p), MYC (Ubp8p) and HA (Gcn5p). The blots shown are representative of three independent experiments. Western blot signals were quantified using the Image J software (NIH), and standard deviations are shown by error bars. ( c ) MYC-tagged wt and rpt2-1 cells were grown in YPD at 30 °C, and total cell extracts were analysed using SDS–PAGE and western blotting using a monoclonal anti-MYC antibody and an anti-ACTIN antibody (control). The quantified results and standard deviations are graphed in the right panel. Western blot signals were quantified using the Image J software (NIH), and standard deviations from four independent experiments are shown by error bars. ( d ) Schematic diagram of in vitro experiments. ( e ) Sgf73-TAP-tagged SAGA complexes purified from wt and rpt2-1 were fractionated by 10–40% glycerol gradient centrifugation, and the fractions were analysed using western blotting with antibodies against CBP (Sgf73p), MYC (Ubp8p) and HA (Gcn5p). IN, input. ( f ) In vitro deubiquitylation assays of three glycerol gradient fractions (fractions 1, 13 and 25) were conducted using HA-ub-FLAG-H2B as the substrate. Western blotting was performed with an antibody against HA. Mock-treated H2Bub1 substrate was used as the input. Full size image In terms of abundance, we observed more Sgf73p and Ubp8p in western blots of Spt7-TAP-purified SAGA complexes from rpt2-1 compared with the wt ( Fig. 2b , lanes 3 and 4). Quantification of the results from three independent experiments ( Fig. 2b , right panel) suggested that the proteasome affects the composition of the SAGA complex in rpt2-1 . We questioned whether this difference in abundance was because of altered expression levels of SAGA components in rpt2-1 ; however, we did not observe any change in the global expression levels of the SAGA complex subunits [20] , [33] , [34] (Sgf73p, Spt20p, Spt8p, Ada1p, Ubp8p, Gcn5p, Ada2p and Sgf11p) in rpt2-1 ( Fig. 2c ). Quantification of the results from three independent experiments supported our conclusion ( Fig. 2c , right panel). Our data suggest that the changes in the SAGA components arise via a post-translational mechanism. As the Sgf73p-Rpt2p interaction was found to trigger the separation of the Sgf73p-Ubp8p-containing complex from the SAGA complex in vitro ( Fig. 1 ), we examined whether this separation occurs through a specific interaction of Sgf73p and Rpt2p in vivo . We performed linear 10–40% glycerol gradient separations of Sgf73-TAP-tagged SAGA complexes purified from wt and rpt2-1 ( Fig. 2d ). After centrifugation, fractions were collected and analysed with the help of western blotting using antibodies against CBP (Sgf73p), HA (Ubp8p) and MYC (Gcn5p) ( Fig. 2e ). The Sgf73p-Ubp8p-containing complex, but not Gcn5p, was detected in fractions 9–15 from the wt samples ( Fig. 2e , top panel). In the rpt2-1 samples, however, Sgf73p and Ubp8p were both absent from fractions 9–15; instead, they were found at the bottom of the gradient (in fraction 25), most likely along with the intact SAGA complexes. These data demonstrate that the proteasome separates the Sgf73p-Ubp8p-containing complex from the SAGA complex both in vitro and in vivo . The DUBm [20] , [21] of the SAGA complex is responsible for deubiquitylating histone H2Bub1 (refs 17 , 18 , 19 ). Owing to the similarities in the composition of the DUBm and the separated Sgf73p-Ubp8p-containing complex, we hypothesized that the dissociated Sgf73p-Ubp8p-containing complex could have deubiquitylation activity. To examine the deubiquitylating ability of the Sgf73p-Ubp8p-containing complex [35] , [36] , [37] , we performed deubiquitylation assays with fractions 1, 13 and 25 from the glycerol gradient assay, using HA-ub-FLAG-H2B as the substrate, and examined the results using western blotting with an antibody against HA. Fraction 13 of the wt samples displayed normal H2Bub1-deubiquitylating activity, whereas that from rpt2-1 did not ( Fig. 2f , compare lanes 4 and 8). Thus, the Sgf73p-Ubp8p-containing complex separated from the SAGA complex has functional deubiquitylation activity. In the SAGA complex, Sgf73p stimulates the deubiquitylation of H2Bub1, and both Sgf73p and Ubp8p are necessary for full DUBm protease activity [35] . This deubiquitylation activity is not only because of the simple dissociation of Ubp8p from the SAGA complex but also involves the release of the Sgf73-DUBm. This finding raises the possibility that the separated complex may be the DUBm of the SAGA complex. As a putative DUBm of the SAGA complex, we designated the dissociated Sgf73p-Ubp8p-containing complex the ‘Sgf73p-DUBm.’ As SAGA is a Gcn5-dependent histone acetyltransferase (HAT) complex [16] , we also employed core histones [38] to examine HAT activity in fractions 1, 13 and 25 ( Supplementary Fig. S2a ) and in purified Spt7-TAP-tagged SAGA complexes from wt and rpt2-1 ( Supplementary Fig. S2b ). Our results revealed that the SAGA complexes of rpt2-1 and wt displayed similar HAT activity levels, indicating that the SAGA complex in the rpt2-1 mutant shows an in vitro histone H3 acetyltransferase activity similar to that of wt . The proteasome shows intact ubiquitin-dependent proteolysis As the altered composition of the SAGA complexes may be because of changes in the proteolytic activity of the proteasome, we assessed the integrity and activity of the 26S proteasome from wt and rpt2-1 . We first examined the molecular integrity of the 19S RP, using purified TAP-tagged-Rpn1p from the wt and rpt2-1 strains. Silver staining showed that the affinity-purified 19S RP complexes from wt and rpt2-1 had nearly identical protein composition patterns ( Fig. 3a ), indicating that the integrity of the 19S RP is maintained in rpt2-1 . 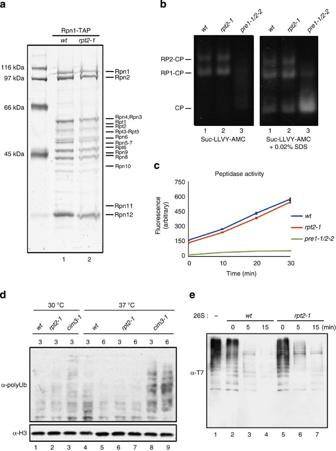Figure 3: The composition of the 19S RP and the proteolytic activity of the 26S proteasome are unaltered inrpt2-1. (a) Rpn1-TAP-tagged 19S RPs fromwtandrpt2-1were purified and visualized using silver staining. Protein molecular weight standards are indicated. (b–c) The 26S proteasomes inrpt2-1show normal peptidase activity and assembly. (b) Purified proteasomes fromwtandrpt2-1were resolved on native gels and stained for hydrolytic activity using the fluorogenic substrate, Suc-LLVY-AMC, in the absence and presence of 0.02% SDS. RP2-CP, RP1-CP and CP refer to doubly capped proteasomes, singly capped proteasomes and the core particle, respectively. (c) Purified proteasomes fromwtandrpt2-1were incubated with the fluorogenic substrate, Suc-LLVY-AMC and peptidase activity was measured with a fluorescence spectrophotometer. Error bars represented standard deviations of three independent experiments. (d) Polyubiquitinated proteins that are not accumulated inrpt2-1.wt,rpt2-1andcim3-1cells were grown to the log phase in YPD at 30 °C and then shifted to 37 °C. The cells were collected at the indicated times, and total cell extracts were subjected to western blotting with FK2 antibodies against polyubiquitin. H3 was used as a control. (e) The 26S proteasome inrpt2-1has intact degradation activity towards polyubiquitinated proteinsin vitro. The 26S proteasomes fromwtorrpt2-1were incubated with polyubiquitinated Sic1PYat 25 °C. The reaction was terminated by the addition of SDS-loading buffer at the indicated times, and the reaction mixture was subjected to western blotting with an antibody against T7. Figure 3: The composition of the 19S RP and the proteolytic activity of the 26S proteasome are unaltered in rpt2-1 . ( a ) Rpn1-TAP-tagged 19S RPs from wt and rpt2-1 were purified and visualized using silver staining. Protein molecular weight standards are indicated. ( b – c ) The 26S proteasomes in rpt2-1 show normal peptidase activity and assembly. ( b ) Purified proteasomes from wt and rpt2-1 were resolved on native gels and stained for hydrolytic activity using the fluorogenic substrate, Suc-LLVY-AMC, in the absence and presence of 0.02% SDS. RP2-CP, RP1-CP and CP refer to doubly capped proteasomes, singly capped proteasomes and the core particle, respectively. ( c ) Purified proteasomes from wt and rpt2-1 were incubated with the fluorogenic substrate, Suc-LLVY-AMC and peptidase activity was measured with a fluorescence spectrophotometer. Error bars represented standard deviations of three independent experiments. ( d ) Polyubiquitinated proteins that are not accumulated in rpt2-1 . wt , rpt2-1 and cim3-1 cells were grown to the log phase in YPD at 30 °C and then shifted to 37 °C. The cells were collected at the indicated times, and total cell extracts were subjected to western blotting with FK2 antibodies against polyubiquitin. H3 was used as a control. ( e ) The 26S proteasome in rpt2-1 has intact degradation activity towards polyubiquitinated proteins in vitro . The 26S proteasomes from wt or rpt2-1 were incubated with polyubiquitinated Sic1 PY at 25 °C. The reaction was terminated by the addition of SDS-loading buffer at the indicated times, and the reaction mixture was subjected to western blotting with an antibody against T7. Full size image To analyse the enzymatic activities of the proteasome, we performed LLVY assays with the fluorogenic substrate, Suc-LLVY-AMC, and purified Rpn1-TAP-tagged 26S proteasomes from wt , rpt2-1 and pre1-1/2-2 (a proteasomal mutant in the beta subunit of the 20S CP and defective in the chymotrypsin-like activity of the 26S proteasome [39] , [40] ). We resolved the affinity-purified 26S proteasome from wt and rpt2-1 on native gels and visualized the active proteasomal complexes using an in-gel activity assay [41] and found that the signal patterns of the ATP-dependent peptidase activities of the proteasomes from wt and rpt2-1 were essentially the same ( Fig. 3b ). We additionally measured the peptidase activity of the proteasome by liquid-based LLVY assays [42] over a time course of 0, 10, 20 and 30 min. Our data showed that the proteasomes purified from wt and rpt2-1 had similar peptidase activities ( Fig. 3c ). These results indicate that the global enzymatic activity and assembly pattern of the proteasome are maintained in the rpt2-1 strain. To examine the ubiquitin-dependent proteolytic function of the 26S proteasome, we assessed polyubiquitinated protein degradation activity in the wt and rpt2-1 strains in vivo ( Fig. 3d ) and in vitro ( Fig. 3e ). We used the proteasome temperature-sensitive ( ts ) mutant, cim3-1 , which is defective in one of the 19S ATPase subunits (Rpt6p) and shows severely reduced proteasome activity at 37 °C (ref. 43 ). wt , rpt2-1 and cim3-1 cells were collected at different times, and total cell extracts were subjected to western blotting with the FK2 antibody against polyubiquitin. Our results revealed that high-molecular-mass polyubiquitinated proteins accumulated to much lower degrees in wt and rpt2-1 cells compared with cim3-1 cells grown at the restrictive temperature ( Fig. 3d , lanes 7–10 versus lanes 11 and 12). Next, using highly polyubiquitinated-Sic1 PY as a substrate [44] , [45] , we performed in vitro measurements of the proteolytic activities of 26S proteasomes purified from wt and rpt2-1 . We found that polyubiquitinated-Sic1 PY was efficiently degraded within 5 min by 26S proteasomes purified from both wt and rpt2-1 ( Fig. 3e , lanes 3 and 6). Thus, the proteasome-mediated degradation of polyubiquitinated proteins does not appear to be defective in the rpt2-1 mutant. The Sgf73-DUBm accumulates near promoter regions in rpt2-1 Our results indicated that the proteasome dissociates the Sgf73-DUBm from SAGA. Therefore, blocking the release of Sgf73-DUBm in rpt2-1 cells is expected to cause retention of Sgf73-DUBm at the sites of SAGA complex recruitment, such as promoters or transcription factor-binding sites. We analysed the relative levels of the Sgf73-DUBm on chromatin in wt and rpt2-1 . We used chromatin immunoprecipitation (ChIP) assays to examine the chromatin association of various SAGA components with the constitutively expressed PMA1 gene in wt and rpt2-1 . Our results revealed that the promoter region of PMA1 was more highly occupied by Sgf73p, Ubp8p and Sgf11p in rpt2-1 versus wt ( Fig. 4a , up to twofold enrichment), whereas the levels of Spt20p, Spt8p, Ada1p, Gcn5p and Ada2p at the promoter and open reading frame (ORF) regions of PMA1 were unaltered or slightly reduced in rpt2-1 compared with the wt ( Supplementary Fig. S3 ). Similar results were obtained from ChIP assays performed with the ADH1 and PYK1 genes ( Fig. 4b,c , and Supplementary Fig. S3 ). These data further confirm that the proteasome affects the composition of SAGA and suggests that intact proteasomes separate the Sgf73-DUBm from the SAGA complex to near promoter regions in wt cells, whereas the undissociated Sgf73-DUBm remains bound to the SAGA complex at promoter regions in rpt2-1 cells. 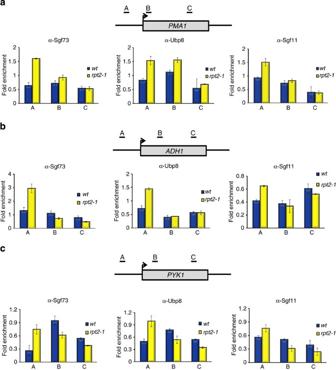Figure 4: The Sgf73p-DUBm shows increased enrichment near the gene promoters inrpt2-1. The relative abundances of Sgf73p, Ubp8p, Gcn5p and Sgf11p on the promoter regions of thePMA1(a),ADH1(b) andPYK1(c) genes inwtandrpt2-1were measured using ChIP assays followed by q-PCR using the indicated primers. ChIP assays and q-PCR were performed on five independent extracts. Standard deviations are shown by error bars. Figure 4: The Sgf73p-DUBm shows increased enrichment near the gene promoters in rpt2-1 . The relative abundances of Sgf73p, Ubp8p, Gcn5p and Sgf11p on the promoter regions of the PMA1 ( a ), ADH1 ( b ) and PYK1 ( c ) genes in wt and rpt2-1 were measured using ChIP assays followed by q-PCR using the indicated primers. ChIP assays and q-PCR were performed on five independent extracts. Standard deviations are shown by error bars. Full size image To examine the effects of rpt2-1 on the recruitment of RNA polymerase II (RNA PolII) to chromatin, we used ChIP to measure the cross-linking of 8WG16 (which detects hypophosphorylated forms of RNA PolII (ref. 46 )) to actively transcribed regions of PMA1 . We observed similar levels of recruitment in wt and rpt2-1 ( Supplementary Fig. S4a ). We also used ChIP analysis to examine the recruitments of the proteasome to the PMA1 gene promoter ( Supplementary Fig. S4b ) and found that the wt and rpt2-1 strains exhibited similar occupancy levels of proteasomal ATPases (for example, Rpt2p and Rpt6p) on the PMA1 promoter regions. Thus, the difference in the recruitment of the SAGA complex to chromatin does not appear to be associated with the recruitment of RNA PolII or the proteasome. Remodelling of SAGA is critical for proper TREX-2 trafficking An association between the TREX-2 (also called THSC) complex and the NPC is critical for the proper export of mRNAs from the nucleus to the cytoplasm, where they are translated into proteins by the cytoplasmic translational machinery [23] , [47] . Previous studies have shown that the interaction between TREX-2 (refs 48 , 49 , 50 , 51 ) and the NPC is mediated by Sgf73p [23] . TREX-2 mediates the association of active genes to the nuclear pores by binding to both the nuclear face of the NPC and the chromatin-bound SAGA complex [52] . As Sgf73p was enriched at the promoter regions in rpt2-1 , we tested whether the separation of the Sgf73-DUBm is important for the trafficking of TREX-2 between chromatin and the NPC. Prior to this analysis, we first examined the integrity of the TREX-2 complex and the SAGA-TREX-2 association in rpt2-1 and observed that these parameters were similar between wt and rpt2-1 ( Supplementary Fig. S5 ). Next, we performed ChIP assays with antibodies against Sac3p and Thp1p to examine the targeting of chromatin-bound TREX-2 to the NPC in the PMA1 genes of the wt , rpt2-1 and sac3Δ strains. Surprisingly, the promoter region of PMA1 was highly occupied by Sac3p and Thp1p in rpt2-1 ( Fig. 5a , up to fourfold and twofold, respectively) compared with the wt . Similar results were obtained from ChIP assays using the ADH1 and PYK1 genes ( Supplementary Fig. S6 ), suggesting that the enrichment of TREX-2 at promoters was not specific to the PMA1 gene. These data demonstrate that the proteasome-mediated remodelling of the SAGA complex is important for the proper association between the TREX-2 complex and the NPC. 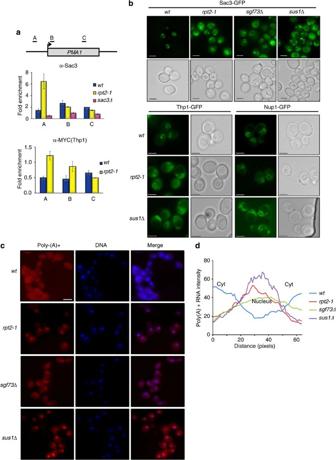Figure 5: Remodelling of the SAGA complex by the Sgf73p-Rpt2p interaction is critical for efficient mRNA export and the TREX-2-NPC associationin vivo. (a) TREX-2 is enriched on the promoter region of thePMA1gene inrpt2-1.ChIP assays of thePMA1gene inwt,rpt2-1andsac3Δwere performed using antibodies against Sac3p and MYC (Thp1p). ChIP assays and q-PCR were performed on five independent extracts. Standard deviations are shown by error bars. (b) The subcellular localization of TREX-2 is affected inrpt2-1. The subcellular localizations of Sac3-GFP, Thp1-GFP and Nup1-GFP inwt,rpt2-1,sgf73Δandsus1Δare shown, as captured using fluorescence microscopy and Nomarski photographs. Scale bar, 5 μm. (c) Export of mRNA is defective inrpt2-1. Analyses of nuclear mRNA export inwt,rpt2-1,sgf73Δandsus1Δare shown. Poly (A)+ RNA was detected using FISH with Cy3-labelled oligo(dT) probes and DNA was stained with 4',6-diamidino-2-phenylindole (DAPI). Scale bar, 10 μm. (d) Quantitative graph of poly-(A)+RNA intensity (assessed using FISH analysis) inwt,rpt2-1,sgf73Δandsus1Δcells is shown. Pairs of cells with nuclei of the same scan width (as determined with DAPI staining) were used for measurements. The cytoplasm (Cyt) and nucleus are indicated. Figure 5: Remodelling of the SAGA complex by the Sgf73p-Rpt2p interaction is critical for efficient mRNA export and the TREX-2-NPC association in vivo . ( a ) TREX-2 is enriched on the promoter region of the PMA1 gene in rpt2-1. ChIP assays of the PMA1 gene in wt , rpt2-1 and sac3Δ were performed using antibodies against Sac3p and MYC (Thp1p). ChIP assays and q-PCR were performed on five independent extracts. Standard deviations are shown by error bars. ( b ) The subcellular localization of TREX-2 is affected in rpt2-1 . The subcellular localizations of Sac3-GFP, Thp1-GFP and Nup1-GFP in wt , rpt2-1 , sgf73Δ and sus1Δ are shown, as captured using fluorescence microscopy and Nomarski photographs. Scale bar, 5 μm. ( c ) Export of mRNA is defective in rpt2-1 . Analyses of nuclear mRNA export in wt , rpt2-1 , sgf73Δ and sus1Δ are shown. Poly (A)+ RNA was detected using FISH with Cy3-labelled oligo(dT) probes and DNA was stained with 4',6-diamidino-2-phenylindole (DAPI). Scale bar, 10 μm. ( d ) Quantitative graph of poly-(A)+RNA intensity (assessed using FISH analysis) in wt , rpt2-1 , sgf73Δ and sus1Δ cells is shown. Pairs of cells with nuclei of the same scan width (as determined with DAPI staining) were used for measurements. The cytoplasm (Cyt) and nucleus are indicated. Full size image As the proteasome-mediated separation of the Sgf73-DUBm from the SAGA complex was found to be important for the TREX-2-NPC interaction, we investigated the subcellular localization of TREX-2 in rpt2-1 using green-fluorescent protein (GFP)-fused Sac3p (the largest component of TREX-2) ( Fig. 5b ). Sac3-GFP was localized predominantly to the nuclear periphery in wt cells ( Fig. 5b , wt ) [23] , but in rpt2-1 and sgf73Δ , it was partly mislocalized to the nuclear periphery and the cytoplasm ( Fig. 5b , rpt2-1 and sgf73Δ ). Furthermore, in the sus1Δ strain, mislocalization of TREX-2 to the cytoplasm was further enhanced ( Fig. 5b , sus1Δ ) [23] . These results indicate that proteasome-mediated remodelling of the SAGA complex is required for the correct targeting of Sac3p to the NPC. Additionally, we analysed the subcellular localization of another TREX-2 component (Thp1p) and a component of the NPC (Nup1p) in rpt2-1 using GFP-fused Thp1p and -Nup1p, respectively. Similar to Sac3-GFP [23] , Thp1-GFP was localized predominantly to the nuclear periphery of wt cells; in rpt2-1 , however, it was partly mislocalized to the nuclear periphery and the cytoplasm. Thus, mislocalization of the TREX-2 complex is not only specific to Sac3p but also correlates with the mislocalization of Thp1p. In contrast, Nup1-GFP was localized to the nuclear side of the NPC in both wt and rpt2-1 cells [53] . These results suggest that the correct targeting of Nup1p to the NPC is unaffected in rpt2-1 . Meanwhile, the sus1Δ strain showed enhanced mislocalization of Thp1-GFP to the cytoplasm but exhibited normal localization of Nup1-GFP. Therefore, the proteasome-mediated remodelling of the SAGA complex does not seem to affect the translocation of nucleoporin to the NPC (that is, the last step of mRNA export). To confirm that rpt2-1 cells are defective in mRNA export, fluorescence in situ hybridization (FISH) analysis was performed using Cy3-labelled oligo (dT) probes ( Fig. 5c , left panel). This analysis revealed a significant accumulation of poly-(A)+ RNA in the nucleus of rpt2-1 cells compared with the wt cells. Deletion of SUS1 was previously shown to trigger significant deficits in mRNA export [50] , whereas deletion of SGF73 induced less accumulation of poly-(A)+ RNA in the nucleus ( Fig. 5c ). Quantification of the nuclear poly-(A)+ RNA intensity levels in wt , rpt2-1 , sgf73Δ and sus1Δ cells ( Fig. 5d ) demonstrated that the proteasome-mediated separation of the Sgf73-DUBm from the SAGA complex is important for efficient mRNA export. rpt2-1 genetically interacts with alleles of Mex67-Mtr2 In the mRNA export pathway, mRNAs form complexes with proteins to generate export-competent ribonucleoparticles [54] that are translocated through the NPC with the help of the Mex67-Mtr2 complex. The Mex67-Mtr2 complex is an essential mRNA export factor that promotes the translocation of ribonucleoparticles by associating with FG repeat nucleoporins [55] . Sac3p interacts directly with Mex67-Mtr2 via these FG repeats [48] and functions in the translocation of Mex67p-Mtr2p through the NPC [51] . In the sac3Δ mutant, the Mex67-Mtr2 complex is mislocalized; this results in synthetic lethality when combined with ts mutants of the Mex67-Mtr2 complex [51] , [56] . Here we investigated the subcellular localization of the Mex67-Mtr2 complex in rpt2-1 using GFP-fused Mex67p and Mtr2p. Mex67p and Mtr2p were found in the nuclear envelope in wt [57] ( Fig. 6a , wt ). In rpt2-1 , however, they were partially mislocalized to the cytoplasm and less significantly to numerous cytoplasmic foci ( Fig. 6a , rpt2-1 ). Therefore, our data indicate that the proteasome-mediated remodelling of the SAGA complex has a direct effect on the proper localization of the Mex67-Mtr2 complex. 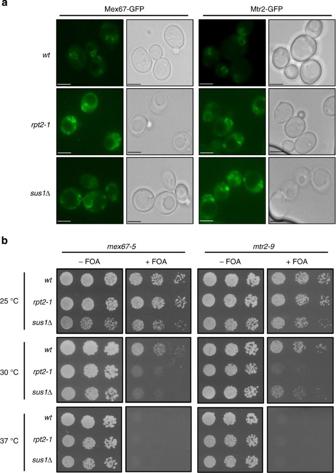Figure 6: The Mex67-Mtr2 complex is mislocalized and interacts genetically with Mex67-Mtr2 mutant alleles inrpt2-1. (a) The subcellular localization of the Mex67-Mtr2 complex is affected inrpt2-1. The subcellular localizations of Mex67-GFP and Mtr2-GFP inwt,rpt2-1andsus1Δare shown, as visualized using fluorescence microscopy and Nomarski photographs. Scale bar, 5 μm. (b) Therpt2-1mutant interacts genetically withmex67-5andmtr2-9. Thetsmutant allelesmex67-5andmtr2-9were transformed into thewt,rpt2-1andsus1Δshuffle strains of wt MEX67 and MTR2 plasmid, respectively. Precultures were diluted in the SC medium and equivalent amounts of cells (1/6 diluted) were spotted on synthetic complete (SC) plates with and without 5-FOA (0.075%).wt MEX67andMTR2plasmids were shuffled out from cells when plated on SC plates with 5-FOA. Plates were incubated for 3 days at 25, 30 and 37 °C. Figure 6: The Mex67-Mtr2 complex is mislocalized and interacts genetically with Mex67-Mtr2 mutant alleles in rpt2-1 . ( a ) The subcellular localization of the Mex67-Mtr2 complex is affected in rpt2-1 . The subcellular localizations of Mex67-GFP and Mtr2-GFP in wt , rpt2-1 and sus1Δ are shown, as visualized using fluorescence microscopy and Nomarski photographs. Scale bar, 5 μm. ( b ) The rpt2-1 mutant interacts genetically with mex67-5 and mtr2-9 . The ts mutant alleles mex67-5 and mtr2-9 were transformed into the wt , rpt2-1 and sus1Δ shuffle strains of wt MEX67 and MTR2 plasmid, respectively. Precultures were diluted in the SC medium and equivalent amounts of cells (1/6 diluted) were spotted on synthetic complete (SC) plates with and without 5-FOA (0.075%). wt MEX67 and MTR2 plasmids were shuffled out from cells when plated on SC plates with 5-FOA. Plates were incubated for 3 days at 25, 30 and 37 °C. Full size image To understand the physiological importance of the rpt2-1 allele in terms of the mRNA export pathway, we asked whether rpt2-1 interacts genetically with other factors involved in mRNA export, such as MEX67 or MTR2 . We used the previously reported 5-fluoro-orotic acid (FOA) screening method to assess synthetic lethality between alleles [56] . We transformed the ts mutant alleles mex67-5 (ref. 56 ) or mtr2-9 (ref. 57 ) into the wt , rpt2-1 and sus1Δ shuffle strains of wt MEX67 or MTR2 plasmid, respectively. We performed spotting assays on plates with or without 5-FOA, and the plates were incubated at 25, 30 and 37 °C. Cells grown on 5-FOA(−) plates showed no apparent growth defects at both permissive and restrictive temperatures. However, cells undergoing plasmid shuffling on 5-FOA(+) plates showed strong ts phenotypes when grown at restrictive temperature: ts phenotypes of mex67-5 and mtr2-9 alleles appeared from all cells grown on 5-FOA(+) at 37 °C (refs 56 , 57 ). In contrast, all mutant cells grown on 5-FOA(+) at 25 °C showed growth pattern similar to wt . Interestingly, double mutants of rpt2-1 with either mex67-5 or mtr2-9 showed significant growth defects compared with wt when grown on 5-FOA(+) at 30 °C ( Fig. 6b ). Furthermore, as demonstrated in a previous study, double mutant of sus1Δ and mex67-5 showed significant growth defects at 30 °C compared with wt on 5-FOA(+) plates [50] . Such enhanced growth retardation on 5-FOA(+) plates indicates synthetic lethality between mex67-5 / mtr2-9 and rpt2-1 alleles. This suggests a strong genetic interaction between rpt2-1 and mRNA export factors MEX67 and MTR2 . Our findings collectively suggest that the proteasome alters the composition of the SAGA complex through the Rpt2p-Sgf73p interaction and that the 19S RP ATP dependently dissociates the Sgf73-DUBm from the SAGA complex in vitro . Previous studies detected Ubp8p at the promoter and ORF regions of GAL1 (ref. 22 ) and showed that Ubp8p interacts specifically with RNA PolII and functions as a component of the SAGA complex at ORFs during transcriptional elongation [20] , [22] . The high occupancy levels of Sgf73p, Ubp8p and Sgf11p at the tested promoter regions in rpt2-1 cells suggest that Ubp8p or the Sgf73-DUBm may have specific roles in transcriptional elongation. It is highly likely that the Sgf73-DUBm of the SAGA complex interacts with ORFs along with phosphorylated RNA PolII and that this is required for transcriptional elongation and is important for the recycling of H2Bub1. Changes in the amount of H2Bub1 in the ORF regions may modulate the uncoupling of SAGA and TREX-2. We found that the total H2Bub1 level was unaltered in the rpt2-1 and SAC3 -deleted strains ( Supplementary Fig. S7 ), suggesting that the distribution of the functional Sgf73-DUBm may be essential for regulating H2Bub1 levels near the ORF. H2B ubiquitylation is required for the efficient reassembly of nucleosomes during transcriptional elongation [58] , [59] , indicating that the Sgf73-DUBm may have an important role in H2Bub1-mediated nucleosome formation and stability. Thus, our findings should contribute to determining the specific links between the chromatin-modifying complex and the nuclear pore/nuclear transport machinery. In addition to their involvement in the remodelling of the SAGA complex, the proteasomal ATPases were found to be critical for efficient mRNA export and the TREX-2-NPC association in vivo . We postulate that the 19S RP-mediated separation of the Sgf73-DUBm is coupled with the mRNA export machinery during transcriptional elongation. The ubiquitylation/deubiquitylation of H2B/H2Bub1 in ORFs may be an important step in the dissociation of the TREX-2 complex from chromatin to the NPC. As Sgf73p recruits the TREX-2 complex to SAGA [23] , the Sgf73-DUBm may help to dissociate TREX-2, allowing it to interact with the NPC. The targeting of SAGA to the promoter and the subsequent ATPase-mediated dissociation of the Sgf73-DUBm link the transcription of mRNA to its export from the nucleus to the cytoplasm ( Fig. 7 ) [60] . Our findings raise the possibility that the proteasome-mediated separation of the chromatin-modifying complex into submodules may be a novel strategy for regulating the intricate patterns of eukaryotic gene expression. 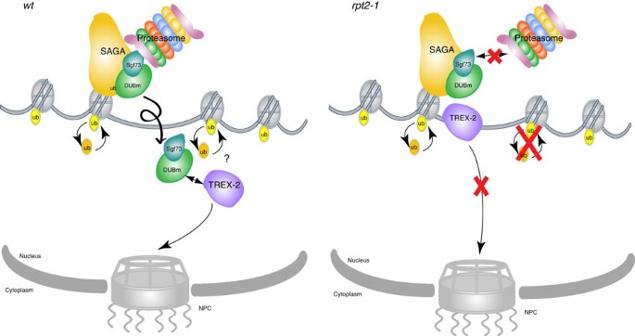Figure 7: Schematic representation of working model. The targeting of SAGA to the promoter and the subsequent dissociation of the Sgf73-DUBm by proteasomal ATPases links H2B ubiquitylation/deubiquitylation to mRNA export. The 19S RP remodels the SAGA complex using the proteasome’s chaperone-like activity, resulting in the formation of a new functional subcomplex of SAGA, which we designated the ‘Sgf73-DUBm’. Upon its dissociation, the Sgf73-DUBm may enter the ORF along with phosphorylated RNA PolII20,22. This is required for transcriptional elongation and is also important for the recycling of H2Bub1. As a result, the TREX-2 complex is dissociated from chromatin and targeted to the NPC by the Sgf73-DUBm. The chaperone-like activity of the proteasome is crucial for mRNA export, as the remodelling of the SAGA complex by the 19S RP is essential for the proper targeting of TREX-2 to the NPC. Therpt2-1strain cannot establish specific binding between the proteasome and SAGA and is thus defective in mRNA export. Figure 7: Schematic representation of working model. The targeting of SAGA to the promoter and the subsequent dissociation of the Sgf73-DUBm by proteasomal ATPases links H2B ubiquitylation/deubiquitylation to mRNA export. The 19S RP remodels the SAGA complex using the proteasome’s chaperone-like activity, resulting in the formation of a new functional subcomplex of SAGA, which we designated the ‘Sgf73-DUBm’. Upon its dissociation, the Sgf73-DUBm may enter the ORF along with phosphorylated RNA PolII [20] , [22] . This is required for transcriptional elongation and is also important for the recycling of H2Bub1. As a result, the TREX-2 complex is dissociated from chromatin and targeted to the NPC by the Sgf73-DUBm. The chaperone-like activity of the proteasome is crucial for mRNA export, as the remodelling of the SAGA complex by the 19S RP is essential for the proper targeting of TREX-2 to the NPC. The rpt2-1 strain cannot establish specific binding between the proteasome and SAGA and is thus defective in mRNA export. Full size image Yeast strains and protein purification All of the strains used in this study are detailed in Supplementary Table S1 . Genomic integration of the C-terminal (TAP, 13MYC, 3HA and GST) and the N-terminal (FLAG) tags and gene deletions were performed using the LiAc/SS-Carrier DNA/PEG method [61] for yeast transformation via homologous recombination of PCR fragments. Yeast cells expressing TAP-tagged protein were grown in Yeast Peptone Dextrose (YPD) at 30 °C to an OD of about 1.0. The cell pellet was resuspended in Lysis buffer (40 mM HEPES (pH 7.5), 350 mM NaCl, 10% Glycerol, 0.1% Tween-20, supplemented with a protease inhibitor) and disrupted using a bead beater (Biospec). Crude whole-cell extracts were subjected to ultracentrifugation, and the supernatant was directly applied to IgG-Sepharose (GE Healthcare) followed by overnight incubation at 4°C with 5 μg of TEV. Three volume of calmodulin-binding buffer (10 mM Tris-Cl, pH 8.0, 1 mM Mg-Ac, 1 mM imidazole, 2 mM CaCl 2 , 0.1% NP-40, 10 mM β-mercaptoethanol, 300 mM KCl and 10% glycerol) was added to the TEV supernatant and incubated with Calmodulin Sepharose (Stratagene) for 3 h. Purified complexes were resolved on 8% SDS–PAGE gels and visualized with silver staining. GST pull-down analysis GST-fusion proteins were bound to glutathione sepharose in PDB (150 mM NaCl, 50 mM HEPES, pH 7.4, 0.1% Tween-20, 10 mM β-mercaptoethanol, 10% glycerol and 1 mM PMSF). The binding reaction was conducted at 4 °C in 0.5 ml of PDB for 1 h. The beads were washed five times in PDB at room temperature, boiled in Laemmli SDS sample buffer (4% SDS, 20% glycerol, 10% β-mercaptoethanol, 0.004% bromophenol blue and 0.125 M Tris-HCl) and resolved using SDS–PAGE. The bound proteins were visualized using western blotting with antibodies against CBP and MYC. In vitro analysis For our in vitro SAGA remodelling assay, 25 μl (~250 ng) of the SAGA complexes from wt and rpt2-1 were incubated in 100-μl reaction volumes containing 5 μl (~1 μg) of the 26S proteasome ( Fig. 1a ) and the 19S RP from wt and rpt2-1 ( Figs. 1b-c ) or the lid and the base complexes from wt ( Fig. 1d ) in reaction buffer (20 mM Tris-HCl, pH 8.0, 25 mM KCl, 5 mM MgCl 2 and 0.01% NP-40 with or without 2 mM ATP) for 1 h at 30 °C with constant mixing. After an additional incubation at 30 °C for 10 min in 300 mM+reaction buffer (20 mM Tris-HCl, pH 8.0, 300 mM KCl, 5 mM MgCl 2 and 0.01% NP-40), 40 μl of calmodulin resin in calmodulin-binding buffer (10 mM Tris-Cl, pH 8.0, 1 mM Mg-Ac, 1 mM imidazole, 2 mM CaCl 2 , 0.1% NP-40, 10 mM β-mercaptoethanol, 300 mM KCl and 10% glycerol) was added to the reaction solution, and resin binding was performed at 4 °C for 2 h. Bead-bound and -unbound (supernatant) proteins were analysed with the help of western blotting on nitrocellulose membranes, using antibodies against CBP (Spt7p) (1:3,000), FLAG (Sgf73p) (1:2,000), MYC (Ubp8p) (1:1,000) and HA (Gcn5p) (1:1,000). The antibodies against CBP (a polyclonal rabbit antibody), HA and MYC (monoclonal mouse antibodies) were produced in-house. The monoclonal mouse anti-FLAG antibody was obtained from Sigma (F1804). Full scans of the western blots are shown in Supplementary Figs S8 and S9 . Deubiquitylation assay The FLAG-tagged ubH2B substrate preparation was modified from a protocol described by Henry et al. [20] Yeast cells expressing FLAG-tagged H2B were grown in YPD at 30 °C to an OD of about 1.0. Cells were collected and washed with 20% trichloroacetic acid (TCA). Cell pellet was resuspended in 0.5 ml of 20% TCA and subjected to vortexing for 2 min with glass beads. The TCA pellet was resuspended in 0.2 ml of 1 X Laemmli sample buffer (2% SDS, 60 mM Tris-HCl, pH 6.8) containing β-mercaptoethanol and unbuffered 2 M Tris. The suspension was boiled for 3 min and centrifuged at 3,000 r.p.m. for 10 min. The supernatant was added to IP buffer (50 mM Tris, pH 7.4, 150 mM NaCl, 0.5% NP-40 and bovine serum albumin (0.5 mg ml −1 )) containing anti-FLAG M2 affinity resin (Sigma). After mixing overnight at 4 °C, the resin was washed with IP buffer. Substrates were eluted by incubation with 2 μl of a 4 mg ml −1 solution of Flag peptide (Kodak) in IP buffer. The 500 ng of substrate was incubated at 37 °C for 5 h in DUB buffer (100 mM Tris-HCl, pH 8.0, 1 mM EDTA, 1 mM dithiothreitol, 5% glycerol, 1 μM PMSF and 1 μg ml −1 pepstatin A) containing 1% of the purified TAP-tagged proteins and various glycerol gradient fractions from wt and rpt2-1 . The reaction was stopped on ice and run on a 16% SDS–PAGE gel. The resolved proteins were transferred to a nitrocellulose membrane, and western blot analysis was conducted using an antibody against HA. LLVY assay The purified proteasome samples were resolved by non-denaturing PAGE, as described in Glickman et al. [62] Briefly, the samples were run on a 3.5% native polyacrylamide gel containing sample dye (xylene cyanol) in a cold room at 100 V for 3.5 h. The gel was then incubated in resolving buffer (90 mM Tris base, 90 mM boric acid, 5 mM MgCl 2 , 0.5 mM EDTA and 1 mM ATP-MgCl 2 ) containing fluorescent peptidase substrate (Suc-LLVY-AMC) with and without 0.02% SDS for 15 min at 30 °C. The proteasome bands were visualized under 380-nm UV light. The liquid-based LLVY assay was performed according to the previously described method [42] . The purified proteasome fractions were tested for peptidase activity with the fluorogenic substrate, Suc-LLVY-AMC, in assay buffer (50 mM Tris-HCl, pH 7.5, 40 mM KCl, 5 mM MgCl 2 , 0.5 mM ATP, 1 mM dithiothreitol). Generation of free AMC was measured and quantified using a fluorescence spectrophotometer (Infinite 200; TECAN) and the Magellan 6 software (Magellan). Assessing the accumulation of polyubiquitinated proteins The wt and rtp2-1 strains were grown in YPD medium at 30 °C to an OD600 of 0.3–0.4 and cultured in YPD at 37 °C. Cells were collected and lysed by the mild alkali method [63] . The extracts were subjected to SDS–PAGE, followed by western blotting with an anti-FK2 antibody (04–263; Millipore) that specifically recognizes polyubiquitin chains [64] . Western blotting was also performed with an anti-H3 antibody (produced in-house) as a control. Polyubiquitinated-Sic1 PY degradation assay The PY motif was introduced into the N-terminal region of Sic1 to generate Sic1 PY , which allows Rsp5 to bind to Sic1. To prepare polyubiquitinated Sic1 PY [65] , mix 1, which is composed of 4.5 μl of buffer A (50 mM Tris-HCl, pH 7.5, 100 mM NaCl, and 10% glycerol), 2 μl of 5 × ATP solution, 0.5 μl of Uba1 (E1), 1 μl of Ubc4 (E4), 2 μl of ubiquitin, was preincubated for 10 min at 25 °C. After preincubation of mix 1, mix 2, which is composed of 6 μl of buffer A, 2 μl of 5 × ATP solution of Rsp5 (E3) and 1 μl of Sic1 PY , was mixed with mix1 and incubated for 3 h at 25 °C. The polyubiquitinated Sic1 PY was incubated with affinity-purified 26S proteasomes from wt and rpt2-1 at 25 °C. The reaction was stopped by the addition of SDS-loading buffer, and the samples were resolved using SDS–PAGE and subjected to western blotting with an anti-T7 antibody (69048-3; Novagen) to assess degradation. Chromatin immunoprecipitation ChIP was performed as previously reported [66] . Yeast cells were grown in YPD at 30 °C to an OD600 of 0.8, followed by cross-linking and sonication. The resulting extracts were immunoprecipitated with antibodies against MYC (a polyclonal rabbit antibody), 8WG16 (ab817; Abcam) and the other indicated proteins (polyclonal rabbit antibodies). Immunoprecipitation was repeated with at least three different extracts per condition. The immunoprecipitated DNA was analysed using quantitative real-time PCR using the CFX96 Real-Time System (Bio-Rad). The cycle thresholds for the target genes were calculated relative to those of the intergenic region on chromosome V. The primers used for PCR are listed in Supplementary Table S2 . Fluorescence imaging and FISH analysis Prior to live-cell imaging, cells were grown to the mid-log phase in YPD ( Figs 5b,c , 6a ). Fluorescence was assessed using an Image M1 fluorescence microscope equipped with a × 100 NA 1.3 oil immersion lens and GFP, 4′,6-diamidino-2-phenylindole dihydrochloride and Cy3 filters (all from Carl Zeiss, Inc.). Images were acquired using an Axio Cam HR camera and the Axio Vision 4.3 software (Carl Zeiss, Inc.) at a resolution of 1,388 × 1,040 (standard mono) at 25 °C. To perform in situ hybridization of poly (A)+ RNA [23] , cells were grown to an OD600 of 0.3–0.4 at 30 °C ( Fig. 5c ) and fixed using 4% paraformaldehyde in 100 mM phosphate buffer (pH 6.5) for 3 h at 25 °C. Cells were added to 0.5 ml of 1.2 M sorbitol in 0.1 M phosphate buffer containing β-mercaptoethanol to form spheroplasts and were incubated for 20 min. Finally, nuclei were counterstained with 0.1 μg ml −1 4′,6-diamidino-2-phenylindole dihydrochloride. How to cite this article: Lim, S. et al. Separation of a functional deubiquitylating module from the SAGA complex by the proteasome regulatory particle. Nat. Commun. 4:2641 doi: 10.1038/ncomms3641 (2013).